Anomalous quantum criticality in an itinerant ferromagnet The dynamics of continuous phase transitions is governed by the dynamic scaling exponent relating the correlation length and correlation time. For transitions at finite temperature, thermodynamic critical properties are independent of the dynamic scaling exponent. In contrast, at quantum phase transitions where the transition temperature becomes zero, static and dynamic properties are inherently entangled by virtue of the uncertainty principle. Consequently, thermodynamic scaling equations explicitly contain the dynamic exponent. Here we report on thermodynamic measurements (as a function of temperature and magnetic field) for the itinerant ferromagnet Sr 1− x Ca x RuO 3 where the transition temperature becomes zero for x =0.7. We find dynamic scaling of the magnetization and specific heat with highly unusual quantum critical dynamics. We observe a small dynamic scaling exponent of 1.76 strongly deviating from current models of ferromagnetic quantum criticality and likely being governed by strong disorder in conjunction with strong electron–electron coupling. SrRuO 3 is a three-dimensional itinerant ferromagnet with the Curie temperature T C ≈160–165 K (refs 1 , 2 , 3 , 4 ). It crystallizes in an orthorhombic perovskite structure with tilted RuO 6 octahedra. In the 4 d 4 configuration of Ru 4+ , the t 2g levels are occupied in a low-spin S =1 state [5] . Ferromagnetism of SrRuO 3 can be suppressed by applying hydrostatic pressure, down to T C ≈50 K at a pressure of 17 GPa [6] . Alternatively, T C is suppressed all the way to absolute zero on substitution of Sr 2+ by the smaller Ca 2+ ions at a critical concentration x c ≈0.7, where Sr 1− x Ca x RuO 3 (SCRO) turns from a ferromagnetic (FM) to a paramagnetic ground state. Whether a quantum critical point (QCP) may be present at x c is a matter of current debate [2] , [4] , [7] , [8] . While specific heat [3] and NMR [4] measurements both concluded that the self-consistent renormalization theory [9] , equivalent to the Hertz–Millis model [10] , [11] , could describe the underlying physics of an FM QCP in SCRO, recent Kerr effect measurements on a composition-spread epitaxial film showed that a possible quantum phase transition (QPT) around a (reduced) critical concentration x c were smeared by disorder originating from the difference of ionic radii between Sr and Ca ions [8] . In addition, on the basis of muon-spin-rotation ( μ SR) experiments, it was argued that a spontaneous phase separation may be a common feature in FM systems near their QPTs, leading to a suppression of dynamic critical behaviour [7] , [12] . From the theoretical point of view, the conventional Hertz–Millis–Moriya model [9] , [10] , [11] predicts, for three-dimensional itinerant magnets, dynamical critical exponents z =2 for antiferromagnets, as well as z =3 for clean and z =4 for disordered ferromagnets [10] . While z =2 has been observed in some antiferromagnets with spin-density-wave order [13] , there are important examples for deviations from the expectation for ferromagnets. Indeed, the model breaks down in the FM case, because extra singular terms arising from fermionic modes, in addition to the order-parameter fluctuations, lead to multiple time scales [14] , [15] , [16] . Moreover, in some composition-driven QPTs, close to the critical concentration x c , disorder effects introduce additional fluctuations, giving rise to a nonanalytic contribution to the free energy between the paramagnetic and locally FM-ordered regions, known as the Griffiths rare regions [17] , [18] , [19] . In the following, we report on a consistent dynamical scaling analysis of the magnetization and specific heat for an x =0.7 sample, bearing all features of a QCP with, however, very unusual critical exponents. In particular, we observe a small dynamic critical exponent z =1.76, which strongly deviates from current models, and may arise from an inhomogeneous electron liquid due to the strong disorder induced by Ca substitution. Magnetic susceptibility and specific heat of Sr 0.3 Ca 0.7 RuO 3 As an overview, we show in Fig. 1a the magnetic d.c. susceptibility χ = M / B , where M is the magnetization and B is the magnetic field, and its reciprocal value χ −1 versus temperature T for 1.8 K≤ T ≤50 K. While χ ( T ) increases with decreasing T down to the lowest temperature of 1.8 K, χ −1 ( T ) shows initially a downward curvature and levels off toward lower T . Notice the gradual change of χ −1 ( T ) from negative to positive curvature with decreasing temperature. The specific heat C ( T ) of Sr 0.3 Ca 0.7 RuO 3 is shown in Fig. 1b in a plot of C / T versus T 2 . Between 20 and 30 K, the specific heat can be described by C / T = γ h + β ph T 2 , where the subscript ‘h’ denotes the extrapolation of C / T from high temperatures to T =0 and β ph T 3 is the usual low- T Debye phonon contribution (see solid line in Fig. 1b ). Below ≈15 K, a positive deviation of C / T from the C / T versus T 2 line is observed with a maximum of C / T for T →0, that is, a zero-temperature cusp. This deviation has been found before and was attributed to spin fluctuations of Ru 4+ moments [3] . However, FM fluctuations should lead to a divergence of C / T at x c for T →0, for example, C / T ∼ log( T 0 / T ). This is not observed in Sr 0.3 Ca 0.7 RuO 3 as will be discussed in more detail below. 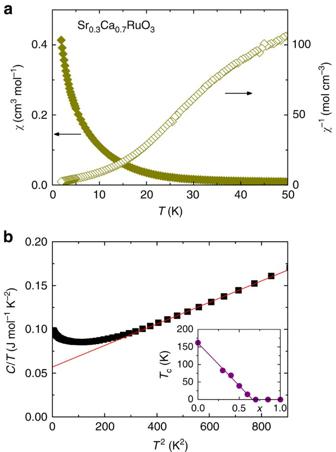Figure 1: Low-temperature magnetic susceptibilityχand specific heatCfor Sr0.3Ca0.7RuO3. (a) Left axis showsχand right axis showsχ−1. The data were measured in the field-cooled mode atB=10 mT. (b) Zero-fieldC/TversusT2. The solid line represents the fit ofC/T=γh+βphT2betweenT=20 and 30 K withγh=0.064 J mol−1K−2andβph=1.3 × 10−4J mol−1K−4. The inset showsTCas a function of Ca concentrationx(ref.21). Figure 1: Low-temperature magnetic susceptibility χ and specific heat C for Sr 0.3 Ca 0.7 RuO 3 . ( a ) Left axis shows χ and right axis shows χ −1 . The data were measured in the field-cooled mode at B =10 mT. ( b ) Zero-field C / T versus T 2 . The solid line represents the fit of C / T = γ h + β ph T 2 between T =20 and 30 K with γ h =0.064 J mol −1 K −2 and β ph =1.3 × 10 −4 J mol −1 K −4 . The inset shows T C as a function of Ca concentration x (ref. 21 ). 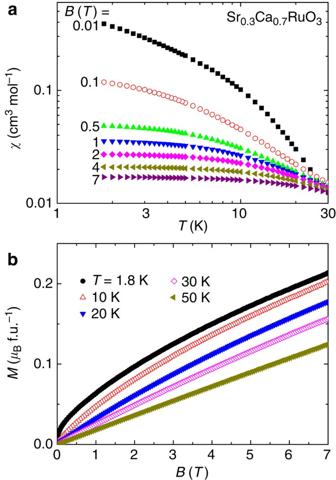Figure 2: Magnetic susceptibilityχand magnetizationMof Sr0.3Ca0.7RuO3. (a) Field-cooledχversus temperatureTmeasured at several different magnetic fields. (b) Magnetic isotherms measured at several different temperatures. Data are shown in part only for clarity. Full size image Figure 2a shows that the magnetic susceptibility χ ( T ) increases more slowly from T =30 to 1.8 K in weak fields. The divergence of χ ( T ) continuously weakens towards lower T , and is increasingly suppressed already in weak magnetic fields. Figure 2b shows that, correspondingly, the magnetic isotherms M ( B ) increase less rapidly with increasing T . The smooth curvatures of χ ( T , B ) and M ( T , B ) suggest the applicability of a scaling relation. We therefore assume that the x =0.7 sample is close to a QCP, see inset of Fig. 1b , as will be substantiated below. Figure 2: Magnetic susceptibility χ and magnetization M of Sr 0.3 Ca 0.7 RuO 3 . ( a ) Field-cooled χ versus temperature T measured at several different magnetic fields. ( b ) Magnetic isotherms measured at several different temperatures. Data are shown in part only for clarity. Full size image Quantum critical scaling of thermodynamic properties At a QCP with hyperscaling, that is, below the upper critical dimension, the scaling relation for the critical part of the free energy reads where b is an arbitrary scale factor and z and βδ / ν are scaling exponents associated with the tuning parameters T and B , respectively. As usual, ν is the correlation length exponent that can be obtained from an analogous scaling relation involving the distance r = x c − x from the critical concentration ( ). δ and β describe the field and concentration dependence of the order-parameter M ( r =0, T =0, B ) ∝ B 1/ δ and M ( r , T =0, B =0) ∝ r β , respectively. For the field and temperature dependence of the magnetization M follows: With the choice of b z T = T 0 with the cutoff energy k B T 0 , we get Hence, M / T β / νz should be a function of B / T βδ / νz . Our data obey the scaling behaviour (Equation (3)). As discussed in the Supplementary Note 1 , the smallest error bars occur when the ratio of the two exponents β / νz and βδ / νz is close to 1.6. This determines the exponent δ ≈1.6 in good agreement with a previous estimate by Itoh et al . [20] To determine the other exponents, we first resort to quantum critical scaling properties of the specific heat that allows an unequivocal determination of d / z and βδ / νz . Then we will return to a discussion of the magnetization data. The scaling behaviour of the critical part of the specific heat is given by Putting again b z T = T 0 yields As long as d > z , this critical contribution at zero field is subleading to the quasiparticle contribution to the specific heat. Nevertheless, equation (5) allows an unequivocal determination of d / z from the zero-field-specific heat, that is, C cr ( T , 0)= T d / z Ψ(0). 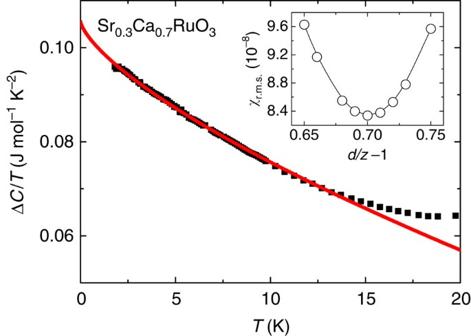Figure 3: Zero-field-specific heat ΔCof Sr0.3Ca0.7RuO3. The phonon contribution has been subtracted. The solid line represents a fit of ΔC/T=γ0−aT0.7between 1.8 and 13 K. The inset shows how the quality of the fit varies with (d−z)/zin equation (5) by checking the smallest mean square deviationχr.m.s.. Figure 3 shows that Δ C / T = C / T − β ph T 2 (with the phonon contribution subtracted) is well described by Δ C / T = γ 0 − aT 0.7 with γ 0 =106 mJ mol −1 K −2 and a =6.0 mJ mol −1 K 2.7 between 1.8 K up to 13 K. Hence, the subleading contribution C cr / T ∝ T 0.7 to the specific heat is clearly visible in the zero-field data. The inset of Fig. 3 displays the root-mean square (r.m.s.) deviation χ r.m.s. versus d / z −1 yielding d / z −1=0.70±0.04 (see Supplementary Fig. 1 ). The striking result following immediately is that the dynamic critical exponent for d =3 is z =1.76±0.04. Figure 3: Zero-field-specific heat Δ C of Sr 0.3 Ca 0.7 RuO 3 . The phonon contribution has been subtracted. The solid line represents a fit of Δ C / T = γ 0 − aT 0.7 between 1.8 and 13 K. The inset shows how the quality of the fit varies with ( d − z )/ z in equation (5) by checking the smallest mean square deviation χ r.m.s. . Full size image Turning to the field dependence of the specific heat, Fig. 4a shows C ( T , B ) plotted as Δ C / T versus log T . With increasing field, the cusp of C / T for T →0 (see Fig. 3 ) becomes rounded and, for B ≥1 T, Δ C / T even falls off slightly towards the lowest measuring temperature. The gradual decrease of Δ C / T from B =0 to 8 T amounts to only 15% in this T range. To check for QCP temperature-field scaling of the specific heat, we plot ( C ( T , B ) − C ( T ,0))/ T d / z versus B / T βδ / νz in Fig. 4b . The zero-field contribution is subtracted to eliminate the non-critical quasiparticle contribution to C . With d / z =1.70 as determined above, we find very good scaling over more than three orders of magnitude in B / T βδ / νz with βδ / νz =1.95±0.1 ( Supplementary Fig. 1 ). The inset of Fig. 4b shows a plot of χ r.m.s. versus the fitting exponent βδ / νz . Due to the small critical contribution to C , the scatter of the scaling plot is somewhat larger. 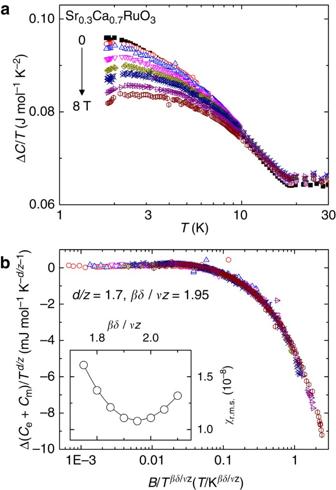Figure 4: Critical contribution to the specific heatC. (a) ΔC(phonon contribution subtracted) of Sr0.3Ca0.7RuO3plotted as ΔC/Tversus logTat fieldsB=0, 0.5, 1, 2, 3, 4, 6 and 8 T from top to the bottom. (b) Scaling of the field-dependent specific heat data from (a). The inset shows how the quality of the scaling collapse varies withβδ/νz(with fixed valued/z=1.7) by checking the smallest mean square deviationχr.m.s.. Figure 4: Critical contribution to the specific heat C . ( a ) Δ C (phonon contribution subtracted) of Sr 0.3 Ca 0.7 RuO 3 plotted as Δ C / T versus log T at fields B =0, 0.5, 1, 2, 3, 4, 6 and 8 T from top to the bottom. ( b ) Scaling of the field-dependent specific heat data from ( a ). The inset shows how the quality of the scaling collapse varies with βδ / νz (with fixed value d / z =1.7) by checking the smallest mean square deviation χ r.m.s. . Full size image Critical scaling of the susceptibility and magnetization We are now in the position to obtain the quantum critical scaling plots for the susceptibility and magnetization data. 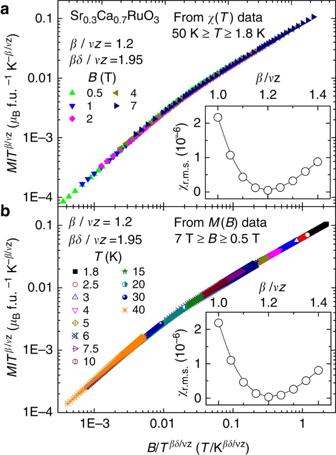Figure 5: Scaling of the magnetic susceptibilityχand magnetizationMas a function of temperatureTand magnetic fieldB. (a) Data fromFig. 2a). (b) Data fromFig. 2b. Insets show how the quality of the scaling collapse varies withβ/νz(with fixed valueβδ/νz=1.95) by checking the smallest mean square deviationχr.m.s.. Figure 5a,b shows the corresponding plots obtained, respectively, from the χ ( T , B ) data of Fig. 2a measured as a function of T for different fields and from the M ( T , B ) data of Fig. 2b measured as a function of B for different temperatures. Here we have omitted the data of very low fields ( B ≤0.1 T of Fig. 2a ) where scaling is not expected because of domain effects. Very good scaling over more than three orders of magnitude of B / T βδ / νz is found for both data sets with β / νz =1.2±0.05 using βδ / νz =1.95 determined from the specific heat ( Supplementary Fig. 2 and Fig. 3 ). Again, the determination of β / νz is corroborated by χ r.m.s. minima shown in the plots of Fig. 5a,b . Our result for β / νz slightly larger than unity is consistent with the experimental observation that T C ( r ) ∝ r νz is roughly proportional to the low- T magnetization ∝ r β (ref. 21 ). The comparatively small value δ =1.63±0.15 that emerges embodies the soft divergence of the susceptibility mentioned earlier. Remember that δ =3 is the mean-field value for the exponent, a value that is usually enhanced via critical fluctuations. Hence, the anomalously small dynamic exponent z obtained from the specific heat results is accompanied by an equally unusual small exponent δ . Using the usual scaling laws, our results further imply a rather large value of the exponent η ≈0.73 that determines the spatial/momentum variation of the susceptibility χ ( q ) ∝ q −(2− η ) and gives evidence for highly non-local quantum fluctuations. Figure 5: Scaling of the magnetic susceptibility χ and magnetization M as a function of temperature T and magnetic field B . ( a ) Data from Fig. 2a ). ( b ) Data from Fig. 2b . Insets show how the quality of the scaling collapse varies with β / νz (with fixed value βδ / νz =1.95) by checking the smallest mean square deviation χ r.m.s. . Full size image The consistent dynamic scaling analysis of magnetization and specific heat of SCRO at the QCP x c =0.7 raises questions to the origin of this highly unusual behaviour. The very observation of scaling of the susceptibility suggests that we are below the upper critical dimension. Together with the numerical value for z , this fact implies that the universality class of the transition cannot be of the conventional type, where d + z >4 would place the system in the mean-field regime. In addition, the negative sign of the critical contribution suggests that one cannot interpret C cr ( T ) as specific heat of isolated collective degrees of freedom but, rather, that the critical dynamics is intertwined with the dynamics of quasiparticles. One possible interpretation is clearly related to the emergence of inhomogeneities. Scale-dependent strain fields, caused by the different values of the ionic radii of Sr and Ca can lead to modified effective exponents [22] . The μ SR relaxation rate T 1 −1 of SCRO for x =0.7 was found to exhibit at low T a behaviour T 1 ∼ constant [12] . A scaling analysis leads to T 1 ∝ T θ with θz =( δ −1) β / ν − d , which for our data yields θ ≅ −1. Given this finding it is important to further experimentally investigate T 1 in the low-temperature regime. The key observation of this paper are the small values of the exponents δ and z , if compared with the mean-field Hertz–Moriya–Millis theory [10] for clean ( δ =3, z =3) or weakly disordered ( δ =3, z =4) systems. Important deviations from mean-field behaviour, based on nonanalytic corrections to Fermi-liquid theory [23] , have been investigated in the vicinity of a ferromagnetic critical point and yield weak first-order transitions [23] , [24] , [25] , instead of fundamentally new critical exponents that are found experimentally in SCRO. Different values for critical exponents have in fact been discussed as a result of the vicinity to a quantum tricritical point [26] or due to preasymtotic critical behaviour in disordered systems [27] . Both approaches yield values for δ rather close to our findings. However, the substantially different value of the dynamical critical exponent found here cannot be explained in refs 26 , 27 . The small value of z seems, however, consistent with a strong-coupling perspective of the coupling between collective magnetic degrees of freedom and incoherent quasiparticle excitations. Away from the critical point, it was shown [28] , [29] that the appropriate description of metallic quantum ferromagnets is in terms of quasiparticles that interact with the coherent magnetization motion via an abelian gauge field. For such a gauge coupling between critical degrees of freedom and the quasiparticle excitations, one would naturally expect a reduced value of the quasiparticle damping and, thus, of the dynamic critical exponent z . Naively, this is due to the fact that in the strong-coupling regime the magnitude of the magnetization is expected to be large even at the QCP, while long-range order is destroyed via directional fluctuations. Hence, the coupling to the Stoner continuum is suppressed by the large magnitude of magnetization, similar to what happens in the ordered state. Our measurement strongly suggests to extend this strong-coupling description of quantum ferromagnetism all the way to the QCP. Regardless of the details, the very observation of dynamic scaling is strong evidence for a second-order transition settling an ongoing debate of this issue [7] . Further work should lead to a detailed understanding of the anomalously low dynamic critical exponent. Sample synthesis and experiments The SCRO polycrystals were prepared by solid-state sintering using SrCO 3 , CaCo 3 and RuO 2 powders as described in ref. 21 . From the structural refinement of powder X-ray diffraction spectra, electron dispersive X-ray spectroscopy and wavelength dispersive X-ray spectroscopy, a stoichiometric single phase (space group Pbnm ) was confirmed. The magnetization M and the specific heat C were measured in the temperature range T =1.8–300 K and in magnetic fields up to B =8 T. We used the same pieces of plate-like samples, with a typical size of 2 × 2 × 1 mm 3 , oriented parallel to the applied field in both measurements. The use of polycrystalline samples does not affect the possibility to reliably determine scaling exponents of phase transitions [21] , yet the concentration dependence of the critical exponents near the classical, finite- T transition is consistent with strain-induced anomalous scaling discussed in ref. 22 , hinting at the role of inhomogeneities. Determination of the critical concentration Since one might wonder whether different values of critical concentration, that is, x c ≠0.7, might lead to a different conclusion on anomalously small dynamic scaling exponent, we further discuss this issue in detail in Supplementary Note 2 . From Supplementary Fig. 4 , x c may be accurate within 3% only. To check the ramifications of this uncertainty, we have additionally carried out a scaling analysis of a sample with x =0.75 ( Supplementary Figs 5 and 6 ). This analysis suggests that while the critical exponents vary slightly when assuming x c =0.75, they are still highly anomalous compared with those of the conventional Hertz–Millis–Moriya model. Using this variation, we show that even if the critical concentration was x =0.65, this would still give anomalous exponents. How to cite this article : Huang, C. L. et al . Anomalous quantum criticality in an itinerant ferromagnet. Nat. Commun. 6:8188 doi: 10.1038/ncomms9188 (2015).